Fine-tuning of auxin homeostasis governs the transition from floral stem cell maintenance to gynoecium formation To ensure successful plant reproduction and crop production, the spatial and temporal control of the termination of the floral meristem must be coordinated. In Arabidopsis , the timing of this termination is determined by AGAMOUS (AG). Following its termination, the floral meristem underdoes gynoecium formation. A direct target of AG, CRABS CLAW ( CRC ), is involved in both floral meristem determinacy and gynoecium development. However, how floral meristem termination is coordinated with gynoecium formation is not understood. Here, we identify a mechanistic link between floral meristem termination and gynoecium development through fine-tuning of auxin homeostasis by CRC. CRC controls auxin homeostasis in the medial region of the developing gynoecium to generate proper auxin maxima. This regulation partially occurs via direct transcriptional repression of TORNADO2 ( TRN2 ) by CRC. Plasma membrane-localized TRN2 modulates auxin homeostasis. We propose a model describing how regulation of auxin homeostasis mediates the transition from floral meristem termination to gynoecium development. The inflorescence meristem undergoes two balanced, antagonistic processes: self-renewal of stem cells to maintain their proliferation activity and recruitment of peripheral cells for organogenesis to form flowers [1] , [2] , [3] . These two mechanisms occur continuously during the reproductive phase. Unlike indeterminate vegetative and inflorescence meristems, floral meristems exhibit a dynamic balance between cell proliferation and organ initiation. Floral meristems sequentially form four types of floral organs without undergoing elongation of the internode between floral organs. Floral meristems are genetically programmed to be terminated at a specific developmental stage after floral organ formation [4] , [5] . Thus, floral meristems are determinate. This precise termination process allows floral meristems to form a female reproductive structure referred to as a gynoecium [6] , [7] . The transcriptional regulatory cascade underlying the termination of floral meristems has been characterized in the model plant Arabidopsis thaliana . Floral meristem termination must be completed during stage 6 of flower development when differential gynoecium growth along the medial-lateral and adaxial-abaxial axis has led to central invagination [8] . The C class gene AGAMOUS ( AG ) plays a central role in this termination process, as well as the establishment of reproductive organ identity [9] , [10] , [11] , [12] . AG turns off the stem cell maintenance program by repressing the expression of the key meristem maintenance gene WUSCHEL ( WUS ) during stage 6 of flower development in a spatio-temporal-specific manner. WUS expression begins to decline when AG is activated [13] , [14] . In ag mutants, WUS expression remains active beyond stage 6, which is sufficient to induce floral meristem indeterminacy [15] , [16] . Temporal WUS repression by AG is controlled by two different pathways. AG is necessary to recruit Polycomb Group protein (PcG) to methylate histone H3K27 at the WUS locus [13] . In addition, WUS repression by AG occurs at least partially through the C2H2 zinc-finger protein KNUCKLES (KNU) [17] . In knu mutants, obvious WUS expression continues after stage 6 in the developing gynoecium [18] . AG directly activates KNU , a process that requires eviction of the PcG complex, leading to cell cycle-dependent KNU induction [18] , [19] . This precise control of KNU activation helps determine the timing of floral meristem termination. After termination of floral meristems, cells located at the center of stage 6 flowers become gynoecium, which consists of two fused carpels [6] , [7] . Previous studies demonstrated that auxin homeostasis contributes to the generation of developmentally important auxin maxima. Not only the well-known PIN-FORMED family of auxin carriers, but also other membrane proteins affect auxin maxima [20] , [21] . For example, TORNADO2 ( TRN2 ) encodes a transmembrane protein of the tetraspanin family, the loss-of-function mutant of which shows aberrant auxin maxima in leaves [22] , [23] , [24] , [25] . In flowers, TRN2 is expressed in stigma at flowers [22] , [24] , [25] . Despite the critical importance of the local action of auxin in gynoecium development, its possible function when floral meristem is terminated is not known. In this study, we obtained insights into a KNU-independent floral meristem termination pathway downstream of AG, which is coordinated by an AG direct target, CRABS CLAW ( CRC ) [26] , [27] , [28] , [29] , [30] , [31] . Previous findings reported that crc knu double mutant shows strong indeterminacy in the floral meristrem [31] and crc mutant phenotype is partially rescued by an auxin transport inhibitor [32] . However, a mechanistic link between floral meristem termination and auxin-mediated gynoecium formation is not known. Here, we found that two direct AG target genes, KNU and CRC , synergistically regulate WUS repression. We further show that CRC represses the expression of TRN2 and controls floral meristem determinacy. Our results highlight the molecular framework underlying the AG-mediated termination of floral meristems through auxin, which is required for subsequent gynoecium development. Indeterminacy in crc knu is caused by WUS misexpression Although CRC is a direct target of AG at stage 6 of flower development [11] , [27] (Supplementary Fig. 1 ), the crc single mutant has only a subtle or no indeterminate floral meristem phenotype [26] . Double mutants in genetic backgrounds with reduced AG expression or with mutations in the downstream target genes of AG show enhanced indeterminacy [29] , [30] , [31] . Because the knu single mutant exhibits an indeterminate phenotype [17] , this mutant provides a sensitized background for studying the role of CRC in floral meristem termination (Supplementary Fig. 2 ). Before conducting a detailed molecular analysis, we confirmed the previously reported aberrant phenotypes of the crc knu double mutant and parental lines [31] (Supplementary Fig. 2a–e ). Compared to the wild type, style tissue is reduced in the crc-1 mutant, leading to the presence of two unfused carpels at the apical region and two separate stigmas ( p = 9.5 × 10 −15 ) (Supplementary Fig. 2a, b, e ). Wild-type and crc-1 mutant fruits contain developing seeds enclosed by carpels (Supplementary Fig. 2a, b ). By contrast, the knu mutants have bulged gynoecia surrounding additional whorls of floral organs (Supplementary Fig. 2c, f ). crc-1 knu-1 double mutant flowers exhibit synergistic indeterminate phenotypes ( p = 9.4 × 10 −14 ) (Supplementary Fig. 2d, e, g ). Although a few fruits showed a weak phenotype without internode elongation, as shown in Supplementary Fig. 2h (categorized as weak crc knu ), most crc knu fruits showed overgrowth of the indeterminate shoot phenotype (categorized as strong crc knu ) (Supplementary Fig. 2d, e, g, i ). This ectopic floral internode axis continued to elongate, with approximately ten rounds of carpel production (Supplementary Fig. 3a ) and stamens occasionally appearing in a spiral pattern (Supplementary Fig. 2i , inset). Due to these phenotypic variations, we divided the mutant phenotypes into five categories based on their phenotypic severity and quantified the phenotypes in this and subsequent analyses (Supplementary Fig. 2e ). To address the role of CRC in floral meristem activity, we monitored the expression of WUS (Fig. 1a–d and Supplementary Fig. 3b–e ). In stage 6 flowers, WUS expression was terminated in wild-type and crc-1 plants (Fig. 1a, b ). In the knu-1 single mutant, weak but distinct WUS signals were detected in the centers of stage 6 and later flowers [18] (Fig. 1a–c and Supplementary Fig. 3b–d ). A strong increase in WUS messenger RNA (mRNA) levels was detected in the crc-1 knu-1 (Fig. 1a–d and Supplementary Fig. 3c–e ). Fig. 1 Indeterminate phenotype of the crc knu double mutant is caused by WUS activity. a – d The floral meristem activity marker WUS mRNA in longitudinal sections of wild-type ( a ) crc-1 ( b ) knu-1 ( c ), and crc-1 knu-1 ( d ) floral buds at developmental stage 6. e – h Flower phenotypes in wus-1 ( e ), wus-1 crc-1 ( f ), wus-1 knu-1 ( g ), and wus-1 crc-1 knu-1 ( h ). i , j Morphology of crc-1 knu-1 ( i ) and wus-1 −/+;crc-1 knu-1 ( j ) fruits. Top: close-up views of fruit tips. Bottom: shapes of whole fruits. Arrowheads indicate stigma structures. Two stigma-like structures were observed in the wus-1 −/+ crc-1 knu-1 mutant due to carpel separation. Images are shown at the same magnification. k Quantification of mutant phenotype. p -values were calculated by χ 2 test ( n = 30). l , m Longitudinal sections of crc-1 knu-1 ( l ) and wus-1 −/+ crc-1 knu-1 ( m ) fruits. Asterisks indicate ectopic carpels. n , o Scanning electron micrographs of fruits with reiterations of floral organs in crc-1 knu-1 ( n ) and wus-1 −/+ crc-1 knu-1 ( o ) fruits. Bars = 50 μm in a – d ; 5 mm in e – h ; 1 cm in i , j bottom; 500 μm in l , m ; and 1 mm in n , o Full size image To investigate whether the observed phenotype depends on the WUS activity, we next created wus-1 crc-1 knu-1 triple mutants to remove WUS activity from the crc knu double mutant. The triple mutant flowers were indistinguishable from those of the wus-1 single mutant (Fig. 1e–h ). These results indicate that wus is epistatic to crc or knu in floral meristems. Furthermore, indeterminacy of the wus-1 −/+ crc-1 knu-1 mutant was significantly rescued compared to the crc-1 knu-1 double mutant ( p = 4.3 × 10 −8 ) (Fig. 1i–o ), suggesting that the indeterminate phenotype of the crc knu mutant is caused by ectopic WUS expression. CRC controls auxin homeostasis and establishes auxin maxima Since synergistic effects are observed in crc knu double mutants, disruption of multiple pathways and drastic transcriptional changes are thought to occur in double mutants, but not in single mutants. To explore the molecular basis for the CRC downstream pathway that affects WUS expression, we performed expression profiling of knu-1 and crc-1 knu-1 . This analysis identified 363 genes whose expression levels were altered more than 2-fold at a 99% confidence level in the crc-1 knu-1 double mutant relative to the knu-1 single mutant (Supplementary Data 1 ). Among those genes, 210 and 153 genes were up- and downregulated in crc knu , respectively (Supplementary Fig. 4a and Supplementary Data 1 ). To investigate the functions of these genes, we performed Gene Ontology (GO) term enrichment analysis using agriGO [33] . GO terms related to numerous metabolic processes were significantly enriched in crc knu ( p < 0.0002, FDR <0.032), and 123 up- or downregulated genes were involved in ‘metabolic processes’ (Fig. 2a , Supplementary Fig. 4b and Supplementary Data 1 and 2 ). To further determine which of the 123 metabolic genes regulate floral meristem determinacy, we determined which genes contained ‘meristem’ in their GO terms (Fig. 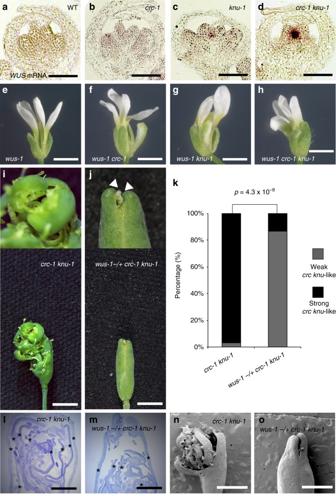Fig. 1 Indeterminate phenotype of thecrc knudouble mutant is caused by WUS activity.a–dThe floral meristem activity markerWUSmRNA in longitudinal sections of wild-type (a)crc-1(b)knu-1(c), andcrc-1 knu-1(d) floral buds at developmental stage 6.e–hFlower phenotypes inwus-1(e),wus-1 crc-1(f),wus-1 knu-1(g), andwus-1 crc-1 knu-1(h).i,jMorphology ofcrc-1 knu-1(i) andwus-1 −/+;crc-1 knu-1(j) fruits. Top: close-up views of fruit tips. Bottom: shapes of whole fruits. Arrowheads indicate stigma structures. Two stigma-like structures were observed in thewus-1 −/+ crc-1 knu-1mutant due to carpel separation. Images are shown at the same magnification.kQuantification of mutant phenotype.p-values were calculated byχ2test (n= 30).l,mLongitudinal sections ofcrc-1 knu-1(l) andwus-1 −/+ crc-1 knu-1(m) fruits. Asterisks indicate ectopic carpels.n,oScanning electron micrographs of fruits with reiterations of floral organs incrc-1 knu-1(n) andwus-1 −/+ crc-1 knu-1(o) fruits. Bars = 50 μm ina–d; 5 mm ine–h; 1 cm ini,jbottom; 500 μm inl,m; and 1 mm inn,o 2b , Supplementary Data 2 and Table 1 ). Among these six genes, two encoded chromatin regulators, CURLY LEAF ( CLF ) and FASCIATA2 ( FAS2 ) [34] , [35] (Fig. 2b ). A ribosomal protein (EMBRYO DEFECTIVE 3105 [EMB3105]), an actin-binding protein (NETWORKED 1A [NET1A]), a HEAT SHOCK PROTEIN 90-like protein (SHEPHERD [SHD]), and a membrane protein (TRN2) were also identified as possible CRC downstream targets [22] , [36] , [37] , [38] (Fig. 2b ). Among these six genes, EMB3105 and TRN2 contained ‘auxin polar transport’ in their GO terms (Fig. 2b and Supplementary Table 1 ). This finding is not unexpected, since metabolic pathways are essential for producing secondary metabolites, including plant hormones [39] . Thus, we hypothesized that a previously hypothesized non-cell-autonomous signal [40] downstream of CRC may be auxin. Fig. 2 Indeterminate phenotype of the crc knu double mutant is rescued by auxin transport inhibitor treatment. a GO terms enriched among the 210 upregulated gene in crc knu . For a list of these genes, see Supplementary Data 1 and 2 . FDR cutoff of <0.03% was implemented. The −log10 adjusted p -values of all significant GO terms are shown. b List of the six genes with likely roles in metabolic process and meristem activity. Among the six genes, EMB3105 and TRN2 play a role in regulating ‘auxin polar transport’, as highlighted in red. c , d Morphology of mock-treated crc-1 knu-1 ( c ) and NPA-treated crc-1 knu-1 ( d ) fruits. Above: close-up views of fruit tips. Below: shapes of whole fruits. Arrowhead indicates stigma structures. e Quantification of mutant phenotype. p -values were calculated by χ 2 test ( n = 30). f , g Longitudinal section of mock-treated crc-1 knu-1 ( f ) and NPA-treated crc-1 knu-1 ( g ) fruits. Asterisks indicate carpels. h , i Scanning electron micrograph of crc-1 knu-1 fruits. h Mock-treated crc-1 knu-1 fruits with several reiterations of floral organs. i NPA-treated crc-1 knu-1 fruits with reduced reiterations. j , k pPIN1::PIN1-GFP expression in wild-type ( j ) and crc-1 ( k ) flowers. l , m In situ hybridization showing the distribution of the adaxial fate marker ARGONAUTE10 ( AGO10 ) in longitudinal sections of wild-type ( l ), and crc-1 ( m ) floral buds at developmental stage 6. n – r DR5rev::3xVENUS expression in wild-type ( n ), mock-treated crc-1 ( o ), NPA-treated crc-1 ( p ), mock-treated crc-1 knu-1 ( q ), and NPA-treated crc-1 knu-1 ( r ) floral buds at developmental stage 6. Insets are closer inspection of floral buds. Arrowheads indicate medial region of gynoecium. Bars = 1 cm in c , d bottom; 500 µm in f , g ; 1 mm in h , i ; 50 μm in j , k and n – o ; and 25 μm in l , m Full size image The style and stigma phenotypes observed in the crc mutant were reportedly rescued by the auxin transport inhibitor N-1-naphthylphthalamic acid (NPA) treatment [32] ( p = 3.4 × 10 −6 ), while wild-type and knu flowers were not significantly affected (Supplementary Figs. 5a –c and 6a–d ). Similar effects were observed when we used 1-naphthoxyacetic acid (1-NOA), which inhibits auxin influx ( p = 3.1 × 10 −7 ) (Supplementary Fig. 5d–f ). This rescue was not observed when we treated the crc mutant with the auxin signaling inhibitor p -chlorophenoxyisobutyric acid (PCIB) (Supplementary Fig. 5g–i ). To further probe the biological importance of the CRC-mediated role of auxin transport in floral meristem determinacy, crc-1 knu-1 plants were treated by inhibitors. NPA and 1-NOA treatments also brought the crc knu double mutant back to the knu mutant phenotype in terms of floral meristem determinacy (NPA: p = 9.4 × 10 −14 ; 1-NOA: p = 6.1 × 10 −13 ), while PCIB did not ( p = 0.31) (Fig. 2c–i and Supplementary Fig. 7a–f ). All of the inner structures in NPA-treated crc-1 knu-1 plants were covered with two carpels, and the number of ectopic carpels was reduced, as observed in the knu-1 mutant (Fig. 2f–i and Supplementary Fig. 6 ). These results suggest that CRC controls auxin transport, but not signaling required for floral meristem termination. We next observed the green fluorescent protein (GFP)-tagged PIN1 line ( pPIN1::PIN1-GFP [41] , [42] , [43] ) to infer possible changes in auxin distribution. In wild-type floral buds at stage 6, PIN1-GFP signals appeared stronger on the medial domain of the gynoecium, which gives rise to the replum, style, and stigma (Fig. 2j ). Basipetal PIN1 polarization caused auxin to move from the top to the bottom of the gynoecium at this stage [43] (Fig. 2k and Supplementary Fig. 8a, b ). Consistent with the slight adaxialization of carpels observed in the crc mutant based on ARGONAUTE10 ( AGO10 ) and PHABULOSA ( PHB ) expression, PIN1 expression domain expanded laterally in the crc mutant, but no difference in its cellular localization was observed (Fig. 2j–m and Supplementary Fig. 8a–d ). Furthermore, no obvious PIN1 expression and localization differences between the wild-type and crc knu mutants were observed at stage 5 flowers prior to floral meristem termination (Supplementary Fig. 8e, f ). By stage 6, the PIN1 expression domain in crc knu was expanded as seen in the crc mutant (Supplementary Fig. 8g, h ). Compared to the wild type, reduced expression of the auxin-response reporter DR5rev::3xVENUS was detected in the crc mutant at the medial domain of the gynoecium [43] (Fig. 2n, o ). Since NPA treatment in crc and crc knu led to increased DR5 signals, phenotypic changes observed in crc and crc knu treated with NPA are likely attributable to enhanced auxin maxima (Fig. 2o–r ). Local auxin production rescues the indeterminacy in crc knu To investigate whether local overproduction of auxin is sufficient to bring crc knu back to knu mutant, we expressed the Agrobacterium indole acetamide (IAM) hydrolase ( iaaH ) gene under the control of the CRC promoter ( pCRC::iaaH ) in these mutants [44] (Fig. 3a–l ). Since iaaH catalyzes the biosynthesis of bioactive auxin (indole-3-acetic acid) from IAM, pCRC::iaaH transgenic plants overproduced auxin in the peripheral region of the floral meristem only when we supplied them with the precursor IAM. In the absence of IAM, the iaaH transgene did not affect mutant phenotypes in either the crc or crc knu mutant background (Fig. 3a, c, e, g, i, k ). Overproduction of auxin by IAM application in the peripheral regions of developing carpels triggered significant rescue of crc mutant phenotypes ( p = 2.2 × 10 −14 ) (Fig. 3m ). IAM-treated pCRC::iaaH fruits exhibited fused carpels (Fig. 3a, b, e, f, i, j ). Likewise, pCRC::iaaH activation also restored the phenotype of the crc knu double mutant to that of knu in terms of floral meristem determinacy ( p = 6.8 × 10 −7 ) (Fig. 3d, h, l, m ). Unlike crc knu double mutants, IAM-treated pCRC::iaaH crc knu plants did not show overgrowth of indeterminate shoots (Fig. 3c, d, g, h, k, l ). By contrast, we did not detect any phenotypic differences in crc or crc knu treated with the optimal concentration of auxin chemicals [45] (Supplementary Figs. 5j –r and 7g–o ), suggesting that auxin maxima may be necessary for proper meristem determinacy. The strong WUS expression observed in crc-1 knu-1 double mutants was attenuated when auxin was locally overproduced (Fig. 3n ). Taken together with the NPA treatment result, our results uncover a possible link between local auxin homeostasis and floral meristem determinacy. Fig. 3 Rescue of crc knu indeterminacy by local overproduction of auxin. a – d Morphology of mock-treated crc-1 pCRC::iaaH ( a ), IAM-treated crc-1 pCRC::iaaH ( b ), mock-treated crc-1 knu-1 pCRC::iaaH ( c ), and IAM-treated crc-1 knu-1 pCRC::iaaH ( d ) fruits. Above: close-up views of fruit tips. Below: shapes of whole fruits. Arrowheads indicate stigma structures. Two stigma-like structures were observed in the mock-treated crc-1 pCRC::iaaH fruits due to carpel separation, while IAM treatment led to carpel fusion. e – h Longitudinal section of mock-treated crc-1 pCRC::iaaH ( e ), IAM-treated crc-1 pCRC::iaaH ( f ), mock-treated crc-1 knu-1 pCRC::iaaH ( g ), and IAM-treated crc-1 knu-1 pCRC::iaaH ( h ) fruits. Asterisks indicate carpels. i – l Scanning electron micrograph of mock-treated crc-1 pCRC::iaaH ( i ), IAM-treated crc-1 pCRC::iaaH ( j ), mock-treated crc-1 knu-1 pCRC::iaaH ( k ), and IAM-treated crc-1 knu-1 pCRC::iaaH ( l ) fruits. m Quantification of mutant phenotypes. Although IAM-treated plants had shorter styles than the controls, we categorized the mutants based on the presence or absence of two stigmatic structures. p -values were calculated by χ 2 test ( n = 30). n mRNA abundance of the stem cell marker WUS , in crc-1 pCRC::iaaH and crc-1 knu-1 pCRC::iaaH flowers with or without IAM. Bars = 1 cm in a – d bottom; 500 µm in e – h ; and 1 mm in i – l Full size image CRC represses TRN2 expression via a YABBY-binding site Based on our expression profiling analysis, we identified two auxin-related targets acting downstream of CRC. Since the role of TRN2 in flower meristem determinacy is largely unknown and the biggest expression changes in crc knu were observed compared knu mutant among six candidate genes (Supplementary Fig. 9a–f ), we focused on the TRN2 gene as a putative direct target of CRC. We first investigated whether CRC regulates TRN2 expression. TRN2 was highly expressed throughout crc-1 carpel primordia at stage 6 compared to wild type (Fig. 4a–c ). Since the TRN2 -misexpressing domain did not fully overlap with CRC (Fig. 4b, c and Supplementary Fig. 9g ), this ectopic expression could be due to the presence of multiple transcriptional activators of TRN2 [25] , feedback regulation via the auxin pathway, and/or lack of mobile signals from YABBY gene activities [46] . Moreover, dexamethasone (DEX) activation of biologically functional and glucocorticoid receptor (GR)-tagged CR protein led to a rapid and reproducible decrease in TRN2 expression (Fig. 4a and Supplementary Fig. 10a ). These results suggest that CRC represses TRN2 expression in stage 6 floral buds. Fig. 4 TRN2 expression is repressed by CRC via a conserved YABBY-binding site. a TRN2 mRNA levels in wild-type and crc-1 flowers (left) and mock- and DEX-treated gCRC-GR (right). p -values were calculated by Student’s t -test ( n = 3). b , c TRN2 mRNA in situ hybridization in longitudinal sections of wild-type ( b ) and crc-1 ( c ) floral buds at developmental stage 6. d Top: pairwise alignment using mVISTA of the upstream intergenic regions of TRN2 from four Brassicaceae species. I, II, and III are conserved regions identified in the TRN2 promoter. Middle: TRN2 promoter structure. Blue bars indicate significant DNase I hypersensitive regions in flowers. Significant regions of DNase I hypersensitive sites were obtained though the Integrated Genome Browser. Bottom: Sequence conservation in the III region of the TRN2 promoter. e Weblogo of YABBY-binding site. f Anti-Myc ChIP in ap1-1 cal-1 35S::AP1-GR after synchronization of flower stages. PCR fragments (TI, TII and TIII, which contain conserved regions) and TRN2 promoter diagram are shown below the ChIP data. Red triangles indicate conserved YABBY-binding site. g , h Reporter expression from wild-type ( g ) and YABBY-binding site-mutated TRN2 promoter ( h ). GUS expression in stage 6 floral buds under the control of the TRN2 promoter with g or without h the YABBY-binding site. i Visual scoring of pTRN2::GUS or pTRN2m::GUS staining in the T1 population; n > 32 for each construct tested. p -values were calculated by Student’s t -test. Bars = 100 µm in b , c ; and 50 µm in g , h Full size image We next attempted to identify cis -regulatory elements important for TRN2 expression. By performing phylogenetic shadowing in four different Brassicaceae species, we identified three conserved regions in the TRN2 promoter (Fig. 4d ). Among these regions, region I and III overlap with DNase hypersensitive sites, where transcription factors can bind [47] . Region III contains a DNase I hypersensitive site only in flowers, where CRC is specifically expressed (Fig. 4d and Supplementary Fig. 10b ). Closer inspection of region III revealed the presence of a previously identified potential YABBY-binding site [48] (GA[A/G]AGAAA) (Fig. 4d, e and Supplementary Fig. 10c ). Chromatin immunoprecipitation (ChIP) analysis using a Myc epitope-tagged CRC protein and floral tissues from flowers that were synchronized in development showed that CRC was specifically enriched at the region TIII containing a conserved site (Fig. 4f ). This result suggests that CRC specifically binds to region III of the TRN2 promoter to repress its transcription in a flower-specific manner, although TRN2 expression in leaves or vasculature is likely regulated by other transcription factor(s) bound by region I of the TRN2 promoter. To investigate whether the YABBY-binding site is necessary for TRN2 expression, we mutagenized this site in the TRN2 promoter, yielding pTRN2m (Fig. 4g–i and Supplementary Fig. 10d–g ). We did not detect the β-glucuronidase (GUS) activity in developing carpels at stage 6 and the reporter was misexpressed when introduced into crc-1 (Fig. 4g and Supplementary Fig. 10h, i ). pTRN2m::GUS was continuously expressed throughout two carpels of stage 6 flowers (Fig. 4g, h ). Increases in pTRN2m :: GUS signals were also detected in sepals, most likely due to the activity of other YABBY family proteins (Fig. 4g, h ). We analyzed the reporter constructs in an independent population of T1 plants ( n ≥ 25) to minimize possible positional effects on transgene expression. Significantly more pTRN2m::GUS lines had stronger signals than pTRN2::GUS lines ( p = 0.005) (Fig. 4i ). These results suggest that a conserved YABBY-binding site is required for proper repression of TRN2 expression. trn2 mutation partially suppresses crc knu To examine whether the floral meristem indeterminacy phenotype in crc knu is caused by the ectopic expression of TRN2 , we eliminated TRN2 activity in the crc knu double mutant (Fig. 5a–i ). The trn2-1 mutant showed reduced TRN2 transcript levels with nonsense mutation [22] and had very small and twisted fruits (Fig. 5a, d, g and Supplementary Fig. 11 ). Two carpels were properly fused in the trn2-1 mutant (Fig. 5a, d, g ). The trn2-1 crc-1 knu-1 mutant exhibited reduced indeterminacy compared to the crc-1 knu-1 parental line ( p = 2.2 × 10 −3 ) (Fig. 5b, c, e, f, h, i, j ). Fig. 5 Removal of TRN2 activity from crc knu partially rescues the floral meristem termination defects in crc knu . a – c Morphology of trn2-1 ( a ), crc-1 knu-1 ( b ), and trn2-1 crc-1 knu-1 ( c ) fruits. d – f Longitudinal sections of trn2-1 ( d ), crc-1 knu-1 ( e ), and trn2-1 crc-1 knu-1 ( f ) fruits. Asterisks indicate carpels. g – i Scanning electron micrographs of trn2-1 ( g ), crc-1 knu-1 ( h ), and trn2-1 crc-1 knu-1 ( i ) fruits. j Quantification of mutant phenotypes. p -values were calculated by χ 2 test ( n = 30). k mRNA abundance of the stem cell marker WUS in trn2-1 , crc-1 knu-1 , and trn2-1 crc-1 knu-1 flowers. l – n WUS mRNA in longitudinal sections of trn2-1 ( l ), crc-1 knu-1 ( m ), and trn2-1 crc-1 knu-1 ( n ) floral buds at developmental stage 6. Images are shown at the same magnification. Bars = 500 µm in a , c , d – f , g – i ; 3 mm in b ; and 100 µm in l – n Full size image We also investigated WUS expression in the triple mutant by both quantitative reverse transcription PCR (qRT-PCR) and in situ hybridization. Consistent with the phenotypic severity, removal of TRN2 activity from crc knu restored WUS mRNA levels to those of trn2-1 (Fig. 5k ). While no WUS mRNA was detected in stage 6 trn2-1 flowers, WUS mRNA levels were very high in crc-1 knu-1 flowers at the same stage. In the trn2-1 crc-1 knu-1 triple mutant, compromised WUS levels were detected compared to crc knu (Fig. 5l–n ). Taken together, these results indicate that WUS repression by CRC is partially dependent on the TRN2 activity. Misexpression of TRN2 in knu mimics crc knu To determine whether TRN2 misexpression is sufficient to mimic the crc mutant phenotype, we expressed TRN2 under the control of the CRC promoter ( pCRC::TRN2 ) (Fig. 6a–d ). pCRC::TRN2 fruits mimicked the crc mutant and no phenotypic difference was observed between pCRC::TRN2 and the crc-1 mutant ( p = 0.15), while the pCRC::TRN2 phenotype differed significantly from the wild type ( p = 4.3 × 10 −13 ) (Fig. 6a, b, e ). We then examined the contribution of TRN2 to the crc-1 knu-1 phenotype by transforming knu-1 plants with pCRC::TRN2 . In contrast to the knu-1 parental line, the pCRC::TRN2 knu-1 plants formed crc knu double mutant-like abnormal fruits bearing extra carpels and stamens due to WUS misexpression (Fig. 6b, c, e, f, h, j–l ). Fig. 6 Ectopic expression of TRN2 mimics the crc mutant phenotype. a – d Morphology of crc-1 ( a ), pCRC::TRN2 ( b ), pCRC::TRN2 knu-1 ( c ), and NPA-treated pCRC::TRN2 knu-1 ( d ) fruits. Top: close-up views of fruit tips. Bottom: shapes of whole fruits. Arrowheads indicate stigma structures. Two stigma-like structures were observed in the crc-1 mutant as well as pCRC::TRN2 due to carpel separation. Images are shown at the same magnification. e Quantification of mutant phenotypes. p -values were calculated by χ 2 test ( n = 30). f , g Longitudinal sections of mock-treated pCRC::TRN2 knu-1 ( f ) and NPA-treated pCRC::TRN2 knu-1 ( g ) fruits. Asterisks indicate carpels. h , i Scanning electron micrograph of pCRC::TRN2 knu-1 fruits with reiterations of floral organs. pCRC::TRN2 knu-1 ( h ) and NPA-treated pCRC::TRN2 knu-1 ( i ) fruits. j – m Floral meristem activity marker, WUS mRNA, in longitudinal sections of crc-1 ( j ), pCRC::TRN2 ( k ), pCRC::TRN2 knu-1 ( l ), and NPA-treated pCRC::TRN2 knu-1 ( m ) floral buds at developmental stage 6. Images are shown at the same magnification. Bars = 1 cm in a – d ; 500 µm in f , g ; 1 mm in h , i ; and 50 µm in j – m Full size image To investigate the link between ectopic TRN2 expression and auxin homeostasis, we treated pCRC::TRN2 lines with NPA. As observed in NPA-treated crc-1 mutants, NPA-treated pCRC::TRN2 plants formed significantly more normal fruits than mock-treated plants ( p = 2.3 × 10 −7 ) (Supplementary Fig. 12a–d ). Moreover, NPA treatment of pCRC::TRN2 knu-1 plants significantly rescued the iteration phenotype ( p = 1.9 × 10 −10 ) (Fig. 6d, e ). Unlike pCRC::TRN2 knu-1 plants, NPA-treated pCRC::TRN2 knu-1 plants produced fused carpels (Fig. 6c–i ). The number of ectopic carpels that formed inside of fruits was reduced, as observed in the knu-1 mutant (Fig. 6f, g and Supplementary Fig. 6c, d, g, h ). In agreement with phenotypic results, qRT-PCR and in situ hybridization showed high levels of WUS expression in pCRC::TRN2 knu plants, but NPA treatment of these plants led to reduced WUS expression (Fig. 6j–m and Supplementary Fig. 12e ). These results suggest that ectopic TRN2 expression is sufficient to mimic the crc mutant phenotype. Plasma membrane-localized TRN2 modulates auxin homeostasis To investigate the function of TRN2, we examined the localization of this protein in reproductive tissues. The gTRN2-GFP transgene we generated rescued the trn2 mutant phenotypes (Supplementary Fig. 13a–f ). TRN2-GFP was mainly detected in the shoot apical meristem and vasculature (Fig. 7a ). Consistent with the finding that TRN2 encodes a transmembrane protein of the tetraspanin family, TRN2-GFP was localized to the plasma membrane (Fig. 7b–d and Supplementary Fig. 13g, h ). We did not detect TRN2-GFP signals in stage 6 carpels, which mimicked the TRN2 promoter expression pattern (Figs. 4 b, g and 7e ). Compared to the wild type, TRN2-GFP protein levels were elevated in the carpel primordia of the crc floral buds at stage 6 (Fig. 7f ). Fig. 7 TRN2 is localized to the plasma membrane and regulates auxin homeostasis. a gTRN2-GFP expression in a wild-type inflorescence. b – d gTRN2-GFP expression ( b ), propidium iodide staining ( c ), and merged ( d ) images of cells in lower part of stage 2 floral primordia. e , f gTRN2-GFP expression in stage 6 floral buds of the wild type ( e ) and crc-1 ( f ). g , h , pPIN1::PIN1-GFP expression in wild-type ( g ) and trn2-1 ( h ) floral buds. i Basipetal IAA transport detection in wild-type and trn2 stem. p -values were calculated by Student’s t -test ( n = 12 for WT, n = 14 for trn2 mutants). j , k DR5rev::3xVENUS expression in wild-type ( j ) and 35S::TRN2- expressing ( k ) Arabidopsis T87 cells. l , m Immunostaining of auxin in wild-type ( l ) and 35S::TRN2- expressing m Arabidopsis T87 cells. n , o DR5rev::3xVENUS expression in wild-type ( n ) and pCRC::TRN2 ( o ) floral buds at stage 6. Insets are closer inspection of floral buds. p Current model for AG-mediated floral meristem termination. Bars = 50 µm in a , e , f , n , o ; 25 µm in g , h , j , k ; and 10 µm in l , m Full size image We next examined PIN1-GFP expression and localization in the trn2 mutant background. In the wild type, PIN1-GFP was highly expressed in the medial domain of the gynoecium (Fig. 7g ). By contrast, PIN1-GFP expression was reduced in trn2 , while the PIN1-GFP expression domain was expanded in crc-1 , in which TRN2 is ectopically expressed (Figs. 2 j, k and 7g, h ). This reduction was not gynoecium-specific, as PIN1-GFP expression in trn2 inflorescences was lower than in the wild type (Supplementary Fig. 13i, j ). We also quantified the transport of radiolabeled IAA in the trn2 mutant grown on MS plates (Supplementary Fig. 13k–n ). This assay showed that trn2 had reduced IAA transport relative to the wild type (Fig. 7i ) ( p = 7.6 × 10 −7 ). Although it was important to ascertain possible roles of TRN2 in auxin transport using trn2 mutants, changes might be simply due to tissue composition issues. To further examine the role of TRN2 in auxin maxima, we compared the DR5 levels in wild-type and 35S::TRN2 cells, including both Arabidopsis T87 cells and tobacco BY-2 cells. We did not observe any differences in terms of cell shape or morphology even if TRN2 was overexpressed in either cell. Regardless of the cells examined, signals from the DR5rev::3xVENUS were reduced in 35S::TRN2 compared to the wild type (Fig. 7j, k and Supplementary Fig. 13o, p ). We also performed immunostaining with auxin antibody using Arabidopsis protoplasts, which allows free auxin to be visualized [49] , [50] , [51] . Based on immunostaining, we detected fewer auxin foci in 35S::TRN2 protoplasts than in untransformed wild-type cells (Fig. 7l, m ). Finally, misexpression of TRN2 under the control of the CRC promoter led to reduced DR5 signals in the medial domain of the gynoecium as seen in crc mutants (Fig. 7n, o ). Taken together, our results suggest that TRN2 modulates auxin homeostasis. Here, we show that the direct AG target CRC controls auxin homeostasis in the developing gynoecium through the negative regulation of TRN2 , thus preventing the overgrowth of floral meristems when KNU is mutated (Fig. 7p ). Two direct AG targets, CRC and KNU , synergistically regulate floral meristem termination, and mutations in these two genes, which act downstream of AG, disrupt the floral meristem determinacy. The confirmation of the striking, synergistic mutant phenotype observed in crc knu sheds light on the importance of these key genes. Synergistic effects triggered by two non-homologous genes are thought to be caused by disruption of multiple or different pathways [52] . Furthermore, strong floral meristem indeterminacy in single crc ortholog mutants has been reported in several other angiosperms [40] . The function of CRC identified in the current study may be conserved during evolution. The AG-WUS and AG-KNU-WUS pathways play central roles in determining the timing of floral meristem termination [13] , [18] , [19] . Precisely how AG alters the activity of a restricted floral stem cell population was previously unknown. Our findings reveal a molecular framework for the spatial regulation of the floral meristem. CRC controls auxin homeostasis partially through TRN2 repression and generates proper auxin maxima to reduce the activity of the floral meristem for subsequent gynoecium formation. In wild-type floral buds at stage 6, auxin maxima as visualized by DR5 expression were observed in the medial domain of the gynoecium. In this domain, auxin maxima are established via regulation of auxin homeostasis, such as auxin transport and local auxin biosynthesis [43] . In crc or crc knu floral buds at stage 6, DR5 expression was greatly reduced. When auxin transport was blocked by auxin transport inhibitors, DR5 expression was recovered in crc or crc knu flowers. Not only NPA treatment, but also local auxin production by iaaH rescued the short style defects in crc and restored the phenotype of the crc knu double mutant to that of the knu mutant in terms of floral meristem determinacy (Supplementary Figs. 5 and 7 ). Since we could not identify any conditions that rescued one of these defects, we favor a model in which changes in auxin homeostasis in the medial regions (including tip of carpels) of the developing gynoecium cause both style and floral meristem determinacy defects. CRC-mediated medial domain initiation through auxin homeostasis during stage 6 of flower development may both turn off floral meristem maintenance and trigger medial domain differentiation, resulting in the formation of the style and the normal tip. Although the pathway that functions downstream of auxin to repress WUS expression is not yet fully understood, one such transcription factor in this pathway has been identified. AUXIN RESPONSE FACTOR3 (ARF3)-mediated auxin perception controls numerous auxin-related events including gynoecium formation [53] , [54] , [55] , [56] ARF3 directly binds to the proximal region of the WUS promoter to repress its expression [57] . Thus, ARF3 might act downstream of the CRC-TRN2 pathway (Fig. 7p ). For decades, molecular and genetic approaches have been used to identify factors that participate in gynoecium development [12] . Numerous tissue-specific transcription factors have been identified [58] . Despite the critical importance of gene regulatory networks regulated by these factors, the downstream target(s) that actually plays a key role in gynoecium formation is currently unknown. Auxin controls gynoecium development [7] , but the genes involved in auxin homeostasis are often expressed throughout the entire plant. Thus, auxin homeostasis must be fine-tuned in a tissue- or stage-specific manner. This study uncovers a molecular link between tissue-specific transcription factors [58] and a gene controlling auxin maxima. AG-activated CRC represses TRN2 , which at least partially controls floral meristem termination. TRN2 expression is correlated with the PIN1 reporter in the carpel primordia at stage 6 of flower development. Both TRN2 and PIN1 proteins were misexpressed in the crc mutant (Figs. 2 j, k and 7e, f ). In contrast, trn2-1 showed reduced PIN1 expression with compromised auxin transport activity (Fig. 7g–i ). Future investigations are needed to understand how TRN2 controls auxin homeostasis. Although the crc mutant phenotype is only seen in flowers, the trn2 mutant shows a pleiotropic phenotype, such as twisted roots or leaves. Thus, CRC seems to act as a flower-specific repressor rather than a general repressor of TRN2 throughout the plant body. Furthermore, TRN2 was misexpressed throughout the carpel, while CRC is only expressed in the abaxial side of carpels. This misexpression could be due to feedback regulation through auxin homeostasis. Alternatives are lack of mobile signals derived from CRC activity, as non-cell-autonomous activities have been reported for all characterized YABBY genes [46] . Since ETHYLENE RESPONSE FACTOR 115 [59] and PSEUDO-RESPONSE REGUALATOR 5 [60] are expressed in carpels [61] and positively regulate TRN2 [25] expression, those activators and CRC might act antagonistically to control TRN2 expression. Since introducing the trn2 mutation into the crc knu double mutant led to only partial phenotypic rescue, TRN2 is not clearly the sole downstream target of CRC in the control of floral meristem termination. Such target(s) might be among the 365 misexpressed genes in crc knu compared to knu . In particular, the final six CRC candidate genes, which are most likely involved in floral meristem termination included SHEPHERD ( SHD ) and CURLY LEAF ( CLF ). Treatment with the auxin transport inhibitor rescued crc knu mutants more thoroughly than did introduction of the trn2 mutation. The different degree of rescue observed in the triple mutants suggests that an auxin-related target might exist that acts directly downstream of CRC and in parallel with TRN2 (Figs. 5 and 7 ). Because our GO term analysis identified many genes involved in metabolic processes (Fig. 2 ), it is also possible that CRC has more downstream targets that jointly control auxin transport and metabolism (biosynthesis, conjugation, and degradation) at multiple levels. Further introducing mutations in CRC candidate target genes into the trn2 crc knu triple mutant would provide insight into the importance of other CRC targets and the CRC downstream pathways for floral meristem determinacy. Genetic stocks and growth conditions All Arabidopsis thaliana seed stocks were in the Landsberg erecta (L er ) background or backcrossed into L er three to four times. The crc-1 [26] , knu-1 [17] , wus-1 [14] , ag-1 35S::AG-GR [62] , ap1-1 cal-5 35S::AP1-GR [63] , pPIN1::PIN1-GFP [41] , and DR5rev::3xVENUS [42] lines were used in this study. For mature plant materials, seeds were sown in pots containing vermiculite and Metro-Mix. For antibiotic selection, plants were grown on Murashige and Skoog (MS) plates. Culture medium consisted of half-strength Murashige and Skoog (MS) salts and 0.8% agar, pH 5.6. All plants were grown at 22 °C under 24-hour light conditions. Phenotypic and statistical analyses The first five fruits from six individual plants (total of 30 fruits) for the wild type and each mutant were categorized into two to five classes based on phenotypic strength. The first five fruits from twenty individual plants (total of 100 fruits) were characterized for Fig. 5j . Plants to be directly compared were grown side-by-side at the same density per pot to minimize potential micro-environmental differences in the growth chamber. Representative images were photographed under an AXIO Zoom.V16 (ZEISS) microscope. Statistical significance was computed using a χ 2 test. Cloning and transformation To construct gCRC-GFP , gCRC-Myc , and gCRC-GR , a genomic fragment covering the 3492 bp region upstream of the CRC translation start site and the 1204 bp coding region were amplified from Landsberg erecta genomic DNA. The resulting DNA fragments were cloned into the binary vectors pGreen0311 (for mGFP) and pGreen0280 (for Myc and GR) and sequenced ( http://www.pgreen.ac.uk ). To construct pCRC::TRN2 or pCRC::iaaH , the 3.5 kbp CRC promoter and coding sequence of TRN2 or iaaH were sub-cloned into pGreen0311 and sequenced. To amplify the iaaH coding sequence, DNA extracted from transgenic plants containing this gene was used as a template. To construct gTRN2-GFP , a genomic fragment covering the 4.1 kb region upstream of the TRN2 translation start site and its coding region was amplified from genomic DNA and cloned into vector pGreen0311. After cloning of these DNA fragments into the pGreen vector, whole functional fragments were transferred into the pENTR 1002 entry vector for the LR reaction; pBGW and pKGW (Invitrogen) were used as destination vectors for the LR reaction. To construct pTRN2::GUS , the 4.1 kbp TRN2 promoter was amplified using gTRN2-GFP as a PCR template and sub-cloned into pENTR/D-TOPO. To mutate the CRC-binding site in the pTRN2 promoter, site-directed mutagenesis was performed using a PrimeSTAR Mutagenesis Basal Kit (Takara) to obtain pTRN2m -pENTR/D-TOPO. After sequencing, the resulting pTRN2 fragments were Gateway-cloned into pGWB3 [64] by the LR reaction. For plant transformation, the inflorescences were dipped in Agrobacterium tumefaciens for 2 min and incubated for 1 day in humid conditions at 4 °C [65] . T1 seeds were collected and screened for antibiotic resistance. More than 20 T1 plants were screened, and representative lines were chosen for further characterization. 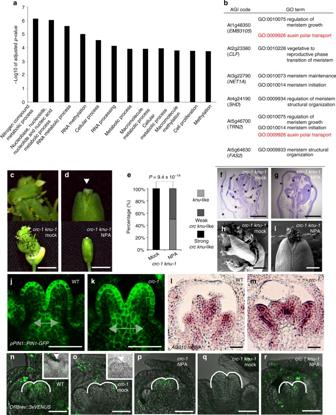Fig. 2 Indeterminate phenotype of thecrc knudouble mutant is rescued by auxin transport inhibitor treatment.aGO terms enriched among the 210 upregulated gene incrc knu. For a list of these genes, see Supplementary Data1and2. FDR cutoff of <0.03% was implemented. The −log10 adjustedp-values of all significant GO terms are shown.bList of the six genes with likely roles in metabolic process and meristem activity. Among the six genes,EMB3105andTRN2play a role in regulating ‘auxin polar transport’, as highlighted in red.c,dMorphology of mock-treatedcrc-1 knu-1(c) and NPA-treatedcrc-1 knu-1(d) fruits. Above: close-up views of fruit tips. Below: shapes of whole fruits. Arrowhead indicates stigma structures.eQuantification of mutant phenotype.p-values were calculated byχ2test (n= 30).f,gLongitudinal section of mock-treatedcrc-1 knu-1(f) and NPA-treatedcrc-1 knu-1(g) fruits. Asterisks indicate carpels.h,iScanning electron micrograph ofcrc-1 knu-1fruits.hMock-treatedcrc-1 knu-1fruits with several reiterations of floral organs.iNPA-treatedcrc-1 knu-1fruits with reduced reiterations.j,kpPIN1::PIN1-GFPexpression in wild-type (j) andcrc-1(k) flowers.l,mIn situ hybridization showing the distribution of the adaxial fate markerARGONAUTE10(AGO10) in longitudinal sections of wild-type (l), andcrc-1(m) floral buds at developmental stage 6.n–rDR5rev::3xVENUSexpression in wild-type (n), mock-treatedcrc-1(o), NPA-treatedcrc-1(p), mock-treatedcrc-1 knu-1(q), and NPA-treatedcrc-1 knu-1(r) floral buds at developmental stage 6. Insets are closer inspection of floral buds. Arrowheads indicate medial region of gynoecium. Bars = 1 cm inc,dbottom; 500 µm inf,g; 1 mm inh,i; 50 μm inj,kandn–o; and 25 μm inl,m Primers used for cloning are listed in Supplementary Table 2 . Chemical treatment For DEX treatment, the inflorescences were sprayed once using 10 μM DEX with 0.01% Silwet for 1 min. The DEX (Sigma) was dissolved in 100% EtOH. Control mock treatment was performed using equal amounts of EtOH with 0.01% Silwet. For RT-PCR, RNA from ag-1 35S::AG-GR and crc-1 gCRC-GR was extracted at 2 and 4 h and only 4 h after DEX treatment, respectively. For ChIP using ap1-1 cal-1 35S::AP-GR , or ap1-1 cal-1 35S::AP1-GR gCRC-myc , the ChIP tissues were fixed 4 days after DEX treatment. For NPA (Tokyo Chemical Industry), 1-NOA (Sigma), PCIB (Sigma), IAA (Wako), NAA (Wako), and 2,4-D (Wako) treatment, 30 μL of 100 μM drugs with 0.01% Silwet was dropped onto the inflorescences of crc-1 , crc-1 knu-1 , pCRC::TRN2 , and pCRC::TRN2 knu-1 plants once when the plant height was ~2 cm. At 6–10 days after treatment, fruit phenotypes were observed. Since all the drugs were dissolved in DMSO, DMSO was used as a mock treatment control. For IAM (Tokyo Chemical Industry) treatment, 10 μM IAM with 0.015% Silwet was dropped onto the inflorescences of pCRC::iaaH crc or pCRC::iaaH crc knu plants for 3 consecutive days when the plant height was ~2 cm. At 6–10 days after treatment, fruit phenotypes were observed. The IAM was dissolved in DMSO. Control mock treatment was performed using equal amounts of DMSO with 0.015% Silwet. Scanning electron microscope To observe the samples by scanning electron microscopy (SEM), tissues were fixed in FAA (45% EtOH, 5% formaldehyde, and 5% acetic acid) overnight at room temperature and dehydrated through a graded ethanol series and acetone. The tissues were critical-point-dried with liquid CO 2 in an HCP-2 critical point dryer (Hitachi) and gold-coated with E-1010 (Hitachi) before SEM imaging. The tissues were imaged under an S-4700 (Hitachi) with an accelerating voltage of 15 kV. More than 10 fruits were observed, and representative images are shown. Sectioning For sectioning, tissues were embedded in Technovit 7100 resin (Heraeus) and polymerized at room temperature overnight. Sections (8 μm thick) were cut with an RM2255 microtome (Leica), dried, stained with 0.05% Toluidine Blue (Wako), mounted on a microscope slide with one or two drops of Mount-Quick (Daido Sangyo), and imaged using an Axio Scope A1 microscope (ZEISS). More than five fruits were sectioned, and representative images are shown. In situ hybridization For in situ hybridization, inflorescences <5 cm long were harvested and fixed in FAA. The resulting tissues were dehydrated in a graded ethanol series, replaced with xylene, and embedded in Paraplast plus (Sigma). Sections (8 µm thick) to be directly compared were processed together. The full length, 5′-UTR and first 472, and 921 bp were used to generate WUS [66] , AGO10 [67] , and PHB [68] probes, respectively. The CRC and TRN2 probes were amplified using cDNA prepared from L er and cloned into the pCRII vector (Invitrogen). In vitro transcription was conducted by T3, T7, or SP6 polymerases. Hybridized tissues were mounted on a microscope slide with one or two drops of Mount-Quick (Daido Sangyo) and observed under an Axio Scope A1 microscope (Zeiss). Two independent experiments were performed, and similar results were obtained. See Supplementary Table 2 for the primers used for in situ probe cloning. GFP observation For GFP observation, confocal laser scanning microscopy (FV1000: Olympus) with objective lens (UPlanSApo: Olympus) was used. Plants 4–8 cm tall that were directly compared were grown side-by-side at the same density per pot to minimize potential micro-environmental differences in the growth chamber. To produce sections of inflorescences, tissues were embedded into 5% agar and sliced with a Liner Slicer PRO7 vibratome (Dosaka). The resulting flower sections were placed onto glasses, mounted on a microscope slide with one or two drops of water or 20 µg/ml PI (Sigma), and observed immediately with an FV1000. The same offset and gain settings were used for all plants for which signal intensity was directly compared. More than five flowers were observed under a confocal microscope, and representative images are shown. Three independent experiments for quantification were performed, and similar results were obtained. The data from one representative experiment are shown. Reverse transcription polymerase chain reaction For RT-PCR, total RNA from floral bud clusters up to stage 10 for mutants [8] or ap1 cal floral bud clusters at 4 h after DEX treatment was extracted using an RNeasy plant mini kit (Qiagen). To remove genomic DNA, an RNase-Free DNase set (Qiagen) was used. The cDNA was synthesized using PrimeScript RT Master Mix (Takara). The cDNA levels were determined with a Light Cycler 480 (Roche) and Light Cycler 480 release 1.5.1.62 SP software (Roche) using FastStart DNA essential DNA Green Master (Roche). The RT-PCR experiments were normalized using the internal control gene EIF4 ( At3g13290 ). The mean and s.e.m. were determined using at least four technical replicates from one representative experiment. Two or three independent experiments were performed, and similar results were obtained. See Supplementary Table 2 for qRT-PCR primers. GUS staining Plant tissue was fixed at room temperature in 90% ice-cold acetone for 15 min, rinsed in GUS staining buffer without 5-bromo-4-chloro-3-indolyl-b-D-glucurinde (X-Gluc), and stained with GUS staining solution (50 mM NaPO 4 , 2 mM K 4 Fe(CN) 6 , 2 mM K 3 Fe(CN) 6 , 2 mM X-Gluc) at 37 °C overnight. The resulting stained tissues were incubated in 70% EtOH for more than 1 week. Plants to be directly compared were grown and stained at the same time. Signal strengths were categorized by visual scoring of independent T1 lines. More than 32 were tested for each construct. Statistical significance was calculated using a Student’s t -test. Tissues were mounted on a microscope slide with one or two drops of chloral hydrate-based clearing solution or 0.05% neutral red (Wako), incubated at room temperature for ~1 h, and imaged using an Axio Scope A1 microscope (Zeiss), AxioCam ERc 5 s camera (Zeiss), and ZEN2 software (Zeiss). Chromatin immunoprecipitation assay To investigate the protein binding of stage-specific transcription factors, ap1-1 cal-1 35S::AP1-GR inflorescences were treated with 10 μM DEX and harvested 4 days later. Inflorescence tissues were fixed with 1% formaldehyde for 15 min, freezed with liquid nitrogen, and kept −80 °C until use. Chromatin was extracted and sonicated to produce DNA fragment under 500 bp. The sonicated DNA was pre-cleared with Protein A beads (Thermo Fisher Scientific) for 2 h at 4 °C. After centrifugation, antibody was added. The tubes were incubated overnight at 4 °C on a rotating device. Beads were then added and incubate for more than 6 h at 4 °C on a rotating device. The resulting beads were washed twice with low salt buffer, high salt buffer, LiCl buffer, and TE buffer. DNA was eluted by incubation for 1 h at 65 °C. Protein-DNA crosslink reversal was conducted overnight at 65 °C. DNA was recovered using QIAquick PCR purification kit (Qiagen). The AG antibody [69] or Myc antibody (9E10; Santa Cruz) was used. The MU gene was used as the negative control locus for ChIP experiments. The ratio of ChIP over input DNA was calculated by comparing the reaction threshold cycle for each ChIP sample to a dilution series of the corresponding input sample and was normalized over mock control loci to obtain fold change. Three independent experiments were performed, and similar results were obtained. The data from one representative experiment are shown. See Supplementary Table 2 for ChIP primers. Gene expression profiling Microarray analysis with three biological replicates was performed with the NimbleGen 12 × 135 K arrays (Roche). The plants were grown at 22 °C under 24-h light conditions. When the plants reached a height of 5–10 cm, inflorescence bud clusters containing flowers of up to stage 10 were harvested. Gene expression was analyzed by Arraystar (DNAStar) with gene annotations from TAIR7. Genes showing a 2.0-fold change in expression within a 99% confidence interval were considered to be differentially expressed and are presented in Supplementary Data 1 . These genes might be involved in various CRC-mediated events, such as floral meristem determinacy, nectary formation, and gynoecium formation. GO term analysis was performed using agriGO software version 1.2 ( http://bioinfo.cau.edu.cn/agriGO/ ). AGI codes from Supplementary Data 1 were used as queries, and all GO terms and hierarchical tree graphs of over-represented GO terms in biological process were downloaded from the agriGO website and are shown in Supplementary Data 2 and Supplementary Fig. 4b , respectively. Phylogenetic shadowing and motif analysis For phylogenetic shadowing, the TRN2 promoter sequences from Arabidopsis halleri (BASO01001507.1), Arabidopsis lyrata (BASP01017915.1), Cannabis sativa (JFZQ01000232.1), and Eutrema salsugineum (AHIU01003814.1) were obtained by NCBI blastn using the Arabidopsis thaliana TRN2 promoter sequence as a query ( http://www.ncbi.nlm.nih.gov/genbank/ ). The promoter sequences were aligned by mVISTA ( http://genome.lbl.gov/vista/mvista/submit.shtml ). Closer inspection of promoter sequences was performed using CLUSTALW ( http://www.genome.jp/tools/clustalw/ ). The sequence logo of cis-elements was generated by WebLogo ( http://weblogo.berkeley.edu ). Culture and transformation of Arabidopsis and tobacco cell lines Tobacco BY-2 and Arabidopsis MM2D cells were cultured in MS medium (4.4 g/L MS salt mix, 30 g/L sucrose, 0.2 g/L 2,4-Dichlorophenoxyacetic acid) at 22 °C in the dark. BY-2/MM2D cells grown on MS agar medium were inoculated into 10 mL of liquid medium and cultured on a rotary shaker at 100 rpm for 1 week. Agrobacterium cells (5 mL at OD600 = 0.8) were washed three times with 5 mL of MS medium (with 250 μg/mL Carbenicillin) and resuspended in 5 mL of MS medium. The 10 mL BY-2/MM2D cell cultures were combined with 100 μL of Agrobacteria in MS and cultured for ~36 h. The BY-2/MM2D cells were then washed four times with MS (with 250 μg/mL Carbenicillin), resuspended in 2 mL of MS, and plated onto MS agar medium. For DR5rev::3xVENUS , the pCR2.1-TOPO vector containing both DR5rev promoter and 3xVENUS-4xAlanine-N7 was used [42] . To generate the 35S::TRN2-GFP construct, eGFP in pGreen with 35S::eGFP-mGFP was replaced by the TRN2 coding sequence. See Supplementary Table 2 for cloning primers. The DR5rev::3xVENUS and 35S::TRN2 constructs were transformed into T87 cells by Agrobacterium tumefaciens (strain C58C1) transformation. The VENUS signals were observed under a Zeiss LSM510 microscope. More than 10 cells were observed, and representative images are shown. 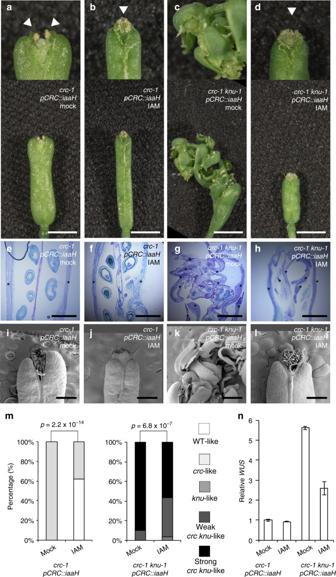Fig. 3 Rescue ofcrc knuindeterminacy by local overproduction of auxin.a–dMorphology of mock-treatedcrc-1 pCRC::iaaH(a), IAM-treatedcrc-1 pCRC::iaaH(b), mock-treatedcrc-1 knu-1 pCRC::iaaH(c), and IAM-treatedcrc-1 knu-1 pCRC::iaaH(d) fruits. Above: close-up views of fruit tips. Below: shapes of whole fruits. Arrowheads indicate stigma structures. Two stigma-like structures were observed in the mock-treatedcrc-1 pCRC::iaaHfruits due to carpel separation, while IAM treatment led to carpel fusion.e–hLongitudinal section of mock-treatedcrc-1 pCRC::iaaH(e), IAM-treatedcrc-1 pCRC::iaaH(f), mock-treatedcrc-1 knu-1 pCRC::iaaH(g), and IAM-treatedcrc-1 knu-1 pCRC::iaaH(h) fruits. Asterisks indicate carpels.i–lScanning electron micrograph of mock-treatedcrc-1 pCRC::iaaH(i), IAM-treatedcrc-1 pCRC::iaaH(j), mock-treatedcrc-1 knu-1 pCRC::iaaH(k), and IAM-treatedcrc-1 knu-1 pCRC::iaaH(l) fruits.mQuantification of mutant phenotypes. Although IAM-treated plants had shorter styles than the controls, we categorized the mutants based on the presence or absence of two stigmatic structures.p-values were calculated byχ2test (n= 30).nmRNA abundance of the stem cell markerWUS, incrc-1 pCRC::iaaHandcrc-1 knu-1 pCRC::iaaHflowers with or without IAM. Bars = 1 cm ina–dbottom; 500 µm ine–h; and 1 mm ini–l Auxin transport assay For basipetal auxin transport assay, the basal 10 mm length of primary inflorescences was used. An inflorescence stem was inserted into a 1.5 ml tube that contained 30 µl of mineral medium and 14 C-IAA (1.8 µM, 3.7 kBq/ml, American Radiolabeled Chemicals, Inc., St. Louis, MO) in the inverted orientation and incubated at 22 °C for 16 h in a humidity chamber. For quantification of 14 C levels, the both apical and basal ends of the stem were cut at the length of 3 mm and were digested by Soluene 350 (Perkin Elmer, Waltham, MA) in capped vials at 50 °C for a day. After the addition of scintillation cocktail (Hionic Fluor, Perkin Elmer, Waltham, MA), the 14 C levels were measured by a liquid scintillation counter (Aloka, Tokyo, Japan). To calculate ratio of basipetal IAA transport, the 14 C levels of the basal side was divided by 14 C levels of the apical side. More than twelve stems were observed for each genotype. Statistical difference was evaluated by Student’s t -test. 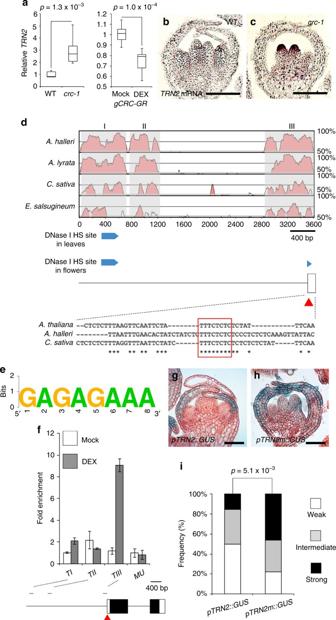Fig. 4 TRN2expression is repressed by CRC via a conserved YABBY-binding site.aTRN2mRNA levels in wild-type andcrc-1flowers (left) and mock- and DEX-treatedgCRC-GR(right).p-values were calculated by Student’st-test (n= 3).b,cTRN2mRNA in situ hybridization in longitudinal sections of wild-type (b) andcrc-1(c) floral buds at developmental stage 6.dTop: pairwise alignment using mVISTA of the upstream intergenic regions ofTRN2from fourBrassicaceaespecies. I, II, and III are conserved regions identified in theTRN2promoter. Middle:TRN2promoter structure. Blue bars indicate significant DNase I hypersensitive regions in flowers. Significant regions of DNase I hypersensitive sites were obtained though the Integrated Genome Browser. Bottom: Sequence conservation in the III region of theTRN2promoter.eWeblogo of YABBY-binding site.fAnti-Myc ChIP inap1-1 cal-1 35S::AP1-GRafter synchronization of flower stages. PCR fragments (TI, TII and TIII, which contain conserved regions) andTRN2promoter diagram are shown below the ChIP data. Red triangles indicate conserved YABBY-binding site.g,hReporter expression from wild-type (g) and YABBY-binding site-mutatedTRN2promoter (h).GUSexpression in stage 6 floral buds under the control of theTRN2promoter withgor withouththe YABBY-binding site.iVisual scoring ofpTRN2::GUSorpTRN2m::GUSstaining in the T1 population;n> 32 for each construct tested.p-values were calculated by Student’st-test. Bars = 100 µm inb,c; and 50 µm ing,h Immunostaining of auxin in BY-2 protoplasts To perform immunostaining, a few droplets of 400 mM mannitol were placed onto the leaves to protect the cells. The tips and petioles of the leaves were removed, and the leaves were cut into strips to facilitate digestion. To digest the cell walls, the leaf strips (or 500 μL of BY-2 cells) were incubated in 3 mL of enzyme solution at room temperature for 3 h with gentle shaking. After incubation, the cells were filtered through a 35–70 μm nylon mesh filter, mixed with 3 mL of pre-chilled W5 buffer, and centrifuged at 100 g for 1 min to collect the cells. 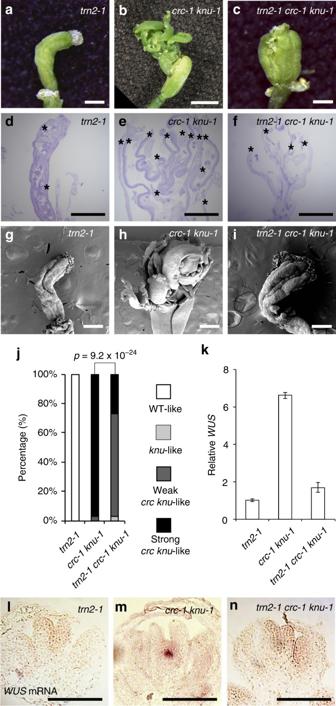Fig. 5 Removal of TRN2 activity fromcrc knupartially rescues the floral meristem termination defects incrc knu.a–cMorphology oftrn2-1(a),crc-1 knu-1(b), andtrn2-1 crc-1 knu-1(c) fruits.d–fLongitudinal sections oftrn2-1(d),crc-1 knu-1(e), andtrn2-1 crc-1 knu-1(f) fruits. Asterisks indicate carpels.g–iScanning electron micrographs oftrn2-1(g),crc-1 knu-1 (h), andtrn2-1 crc-1 knu-1(i) fruits.jQuantification of mutant phenotypes.p-values were calculated byχ2test (n= 30).kmRNA abundance of the stem cell markerWUSintrn2-1,crc-1 knu-1, andtrn2-1 crc-1 knu-1flowers.l–nWUSmRNA in longitudinal sections oftrn2-1(l),crc-1 knu-1(m), andtrn2-1 crc-1 knu-1(n) floral buds at developmental stage 6. Images are shown at the same magnification. Bars = 500 µm ina,c,d–f,g–i; 3 mm inb; and 100 µm inl–n 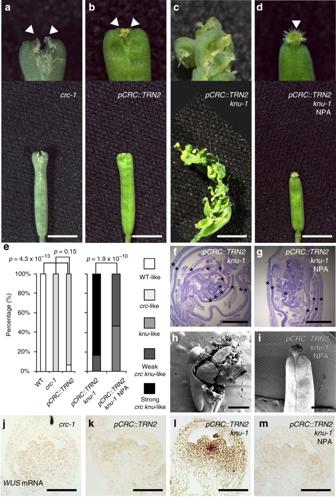Fig. 6 Ectopic expression ofTRN2mimics thecrcmutant phenotype.a–dMorphology ofcrc-1(a),pCRC::TRN2(b),pCRC::TRN2 knu-1(c), and NPA-treatedpCRC::TRN2 knu-1(d) fruits. Top: close-up views of fruit tips. Bottom: shapes of whole fruits. Arrowheads indicate stigma structures. Two stigma-like structures were observed in thecrc-1mutant as well aspCRC::TRN2due to carpel separation. Images are shown at the same magnification.eQuantification of mutant phenotypes.p-values were calculated byχ2test (n= 30).f,gLongitudinal sections of mock-treatedpCRC::TRN2 knu-1(f) and NPA-treatedpCRC::TRN2 knu-1(g) fruits. Asterisks indicate carpels.h,iScanning electron micrograph ofpCRC::TRN2 knu-1fruits with reiterations of floral organs.pCRC::TRN2 knu-1(h) and NPA-treatedpCRC::TRN2 knu-1(i) fruits.j–mFloral meristem activity marker,WUSmRNA, in longitudinal sections ofcrc-1(j),pCRC::TRN2(k),pCRC::TRN2 knu-1(l), and NPA-treatedpCRC::TRN2 knu-1(m) floral buds at developmental stage 6. Images are shown at the same magnification. Bars = 1 cm ina–d; 500 µm inf,g; 1 mm inh,i; and 50 µm inj–m 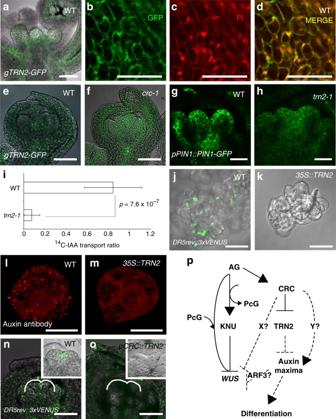Fig. 7 TRN2 is localized to the plasma membrane and regulates auxin homeostasis.agTRN2-GFPexpression in a wild-type inflorescence.b–dgTRN2-GFPexpression (b), propidium iodide staining (c), and merged (d) images of cells in lower part of stage 2 floral primordia.e,fgTRN2-GFPexpression in stage 6 floral buds of the wild type (e) andcrc-1(f).g,h,pPIN1::PIN1-GFPexpression in wild-type (g) andtrn2-1(h) floral buds.iBasipetal IAA transport detection in wild-type andtrn2stem.p-values were calculated by Student’st-test (n= 12 for WT,n= 14 fortrn2mutants).j,kDR5rev::3xVENUSexpression in wild-type (j) and35S::TRN2-expressing (k)ArabidopsisT87 cells.l,mImmunostaining of auxin in wild-type (l) and35S::TRN2-expressingmArabidopsisT87 cells.n,oDR5rev::3xVENUSexpression in wild-type (n) andpCRC::TRN2(o) floral buds at stage 6. Insets are closer inspection of floral buds.pCurrent model for AG-mediated floral meristem termination. Bars = 50 µm ina,e,f,n,o; 25 µm ing,h,j,k; and 10 µm inl,m The cells were washed once, resuspended in cold W5 buffer, and incubated for 30 min on ice. After incubation, the cells were centrifuged at 100 g for 1 min and resuspended in 300 μL of W6 buffer. A circle was drawn on ProbeOn glass slides with a PAP pen. The 300 μL cell suspension was dropped onto the circle, and the slide was incubated for 1 h to allow the cells to adhere to the slide. The W6 buffer was carefully removed, and the cells were fixed with fixing solution (4% formaldehyde in W6 solution) and incubated for 1 h at room temperature. The cells were washed three times with 300 μL of TSW buffer for 10 min per wash for permeabilization, followed by incubation with primary antibody [49] , [50] , [51] (anti-auxin) (Sigma-Aldrich) diluted in 300 μL of TSW buffer at 4 °C for 16 h in a moist chamber. The samples were washed three times with 300 μL of TSW buffer for 10 min per wash to remove the unbound antibody, followed by incubation with secondary antibody diluted in 300 μL of TSW buffer at room temperature for 3 h. After three additional washes with 300 μL of TSW buffer for 10 min per wash to remove the unbound secondary antibody, the samples were mounted with 70 μL of DAPI, covered with a coverslip, and sealed with clear nail polish for longer storage. The VENUS signals were observed under a Zeiss LSM510 microscope. The VENUS signals were observed under a Zeiss LSM510 microscope. More than 10 cells were observed, and representative images are shown. Data availability The data that support the findings of this study are available from corresponding author on request. The microarray data have been deposited in GEO under accession number GSE88969.